Species traits and phylogenetic conservatism of climate-induced range shifts in stream fishes Understanding climate-induced range shifts is crucial for biodiversity conservation. However, no general consensus has so far emerged about the mechanisms involved and the role of phylogeny in shaping species responses has been poorly explored. Here, we investigate whether species traits and their underlying phylogenetic constraints explain altitudinal shifts at the trailing and leading edges of stream fish species ranges. We demonstrate that these shifts are related to dissimilar mechanisms: whereas range retractions show some support for phylogenetic clustering due to a high level of conservatism in thermal safety margins, range expansions are underpinned by both evolutionarily conserved and labile traits, notably trophic position and life-history strategy, hence decreasing the strength of phylogenetic signal. Therefore, while climate change brings many difficulties in establishing a general understanding of species vulnerability, these findings emphasize how combining trait-based approaches in light of the species evolutionary history may offer new opportunities in facing conservation challenges. Evidence is accumulating that ongoing climate change is causing many species to shift their geographic ranges drastically so as to remain within their ancestral environment (that is, niche-tracking) [1] , [2] . Throughout their evolutionary (that is, phylogenetic) history, species have been continuously exposed to climate fluctuations. Since species traits influenced by climate generally exhibit a phylogenetic pattern whereby closely related species share similar traits [3] , [4] , climate changes in the past have resulted in lineage-specific extinction rates [5] , [6] . However, how the evolutionary history of species constrains their ability to track niches has been poorly assessed and determining the characteristics that underlie species sensitivity and/or vulnerability to contemporary climate change remains crucial for the development of effective conservation and management strategies [7] , [8] . Present-day geographical biodiversity patterns have been strongly shaped by two distinct processes affecting range dynamics: the expansions and contractions caused by Pleistocene glacial-interglacial cycles [9] , [10] . As a result, population dynamics at the edges of the distribution range are critical in determining the vulnerability of species to changing climate and, ultimately, for their long-term persistence: colonization by leading populations (that is, cold limits at high elevation and latitude) [2] , [11] and extirpation of trailing populations (warm limits at low elevation and latitude) [12] , [13] . Idiosyncratic responses of species to climate change are underpinned by the interplay between three dimensions of climate change vulnerability, namely exposure (the extent to which the species thermal habitat changes), intrinsic sensitivity (for example, due to physiological limits or trophic specialization) and resilience capacity (species ability to avoid negative impacts of climate change through dispersal and/or microevolutionary or phenotypic changes) [14] , [15] . Several biological, physiological and ecological traits may thus be involved ( Fig. 1 ), although we still know little about the mechanisms underlying the complex nature of range shifts [16] . Despite recent advances [7] , there is no general consensus about the effects of species traits on range expansion, while the mechanisms driving the response of trailing populations have so far been poorly explored [17] , [18] . Identifying the phylogenetic signal in range shifts may help decipher the mechanisms underlying differences in how species respond to climate change [19] . Conservatism of range shifts at the leading and trailing edges of distribution can be expected to be driven by the degree of phylogenetic clustering of traits involved in responding to climate change [5] . 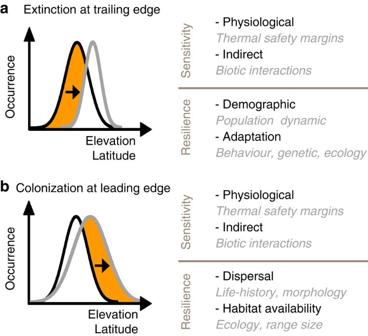Figure 1: Theoretical expectations about the underlying mechanisms of range shifts in ectotherms. Contemporary climate change is driving widespread (a) extinction at the trailing edge and (b) colonization at the leading edge, resulting in range shifts upslope and polewards1,2. Ectotherms are especially sensitive to climate change, because their physiology is directly influenced by temperature. Thermal preferences coincide with temperatures that maximize fitness, and individual performance rapidly drops outside the optimal range22,25. The impact of warming, however, depends on the covariations of fitness curves and regional climate23,25. The thermal safety margins, describing the warming tolerance of organisms relative to their current thermal habitat, should thus be the principal trait driving extinctions or shifts to cooler habitats20,21. These effects could also be indirect, since climate change modifies the architecture of food webs as a result of the differing thermal sensitivities of interacting species12,20. Additional traits underlying the ability of species to respond to climate change impacts (that is, resilience ability) may, however, delay extinction at the trailing edge or impede colonization at the leading edge, although acting in opposite directions8,65. At the trailing edge, where thermal physiology or biotic interactions limit range-edge populations, even a small degree of warming could have major consequences22,25. Given the rate and magnitude of changes in climate, these populations may have a limited capacity to cope with new climatic conditions4,66. Nevertheless, propagule pressure (that is, the quantity and frequency of dispersing individuals) may enable species to temporarily compensate for local extinctions caused by adverse climatic conditions55,65. Alternatively, thermal stress can be buffered through adaptation, acclimatization and/or behavioural adjustments22,23, so that the extinction risk may be greater for environmentally specialized species, and especially significant for range-restricted species4. At the leading edge, dispersal limitations can prevent range expansion since successful colonization relies on the propensity to disperse, the ability to disperse, and the establishment of propagules outside the current species distribution26. A wide range of traits may be involved, including mobility, propagule pressure, environmental requirements (for example, resource and habitat specialization) and geographical range of species9,26,55. Figure 1: Theoretical expectations about the underlying mechanisms of range shifts in ectotherms. Contemporary climate change is driving widespread ( a ) extinction at the trailing edge and ( b ) colonization at the leading edge, resulting in range shifts upslope and polewards [1] , [2] . Ectotherms are especially sensitive to climate change, because their physiology is directly influenced by temperature. Thermal preferences coincide with temperatures that maximize fitness, and individual performance rapidly drops outside the optimal range [22] , [25] . The impact of warming, however, depends on the covariations of fitness curves and regional climate [23] , [25] . The thermal safety margins, describing the warming tolerance of organisms relative to their current thermal habitat, should thus be the principal trait driving extinctions or shifts to cooler habitats [20] , [21] . These effects could also be indirect, since climate change modifies the architecture of food webs as a result of the differing thermal sensitivities of interacting species [12] , [20] . Additional traits underlying the ability of species to respond to climate change impacts (that is, resilience ability) may, however, delay extinction at the trailing edge or impede colonization at the leading edge, although acting in opposite directions [8] , [65] . At the trailing edge, where thermal physiology or biotic interactions limit range-edge populations, even a small degree of warming could have major consequences [22] , [25] . Given the rate and magnitude of changes in climate, these populations may have a limited capacity to cope with new climatic conditions [4] , [66] . Nevertheless, propagule pressure (that is, the quantity and frequency of dispersing individuals) may enable species to temporarily compensate for local extinctions caused by adverse climatic conditions [55] , [65] . Alternatively, thermal stress can be buffered through adaptation, acclimatization and/or behavioural adjustments [22] , [23] , so that the extinction risk may be greater for environmentally specialized species, and especially significant for range-restricted species [4] . At the leading edge, dispersal limitations can prevent range expansion since successful colonization relies on the propensity to disperse, the ability to disperse, and the establishment of propagules outside the current species distribution [26] . A wide range of traits may be involved, including mobility, propagule pressure, environmental requirements (for example, resource and habitat specialization) and geographical range of species [9] , [26] , [55] . Full size image Previous studies have claimed that thermal sensitivity of species might be the main trait shaping vulnerability [20] , [21] , [22] . In that case, range contraction at the trailing edge is expected to be phylogenetically clustered as thermal tolerances are generally strongly conserved along the phylogeny [3] , [4] . A number of recent analyses [23] , [24] , [25] have demonstrated, however, that potential consequences of climate change depend both on the temperature dependence of fitness but also on the position of species relative to local climate. Biotic interactions or traits promoting local persistence may also enhance the variability of temperature-dependent extinction to a certain extent ( Fig. 1 ). In contrast, colonization at the leading edge should strongly depend on multiple dispersal and establishment traits that are subjected to various selection pressures. The influence of dispersal limitation on range expansion may ultimately lead to decreasing phylogenetic signal expected from the thermal sensitivity of species [26] , [27] . Indeed, morphological traits linked to dispersal ability (for example, mobility through body size) are commonly conserved along the phylogeny, whereas several behavioural and ecological traits related to establishment success (for example, degree of habitat specialization should decrease habitat available for the species) are thought to be more evolutionarily labile [28] , [29] . Consequently, we expected to find little or no phylogenetic clustering of range expansion at the leading edge. As far as we are aware, however, the effect of evolutionary constraints on how species track shifting climate has so far remained largely unexplored. Here, we used range shifts documented for stream fish to assess whether phylogenetic patterns in shifts at the leading and trailing edges along an altitudinal gradient resulted from conservatism of the traits involved in species response to climate change. Stream fishes provide ideal model organisms for studying climate-induced range shifts because of their ectothermic physiology, relatively short generation times and constrained distribution within hydrographic networks, thus promoting directional shifts. Specifically, we aimed (i) to test whether range-shifting species were phylogenetically more closely related than would be expected by chance and (ii) to confront several non-exclusive theoretical expectations ( Fig. 1 ) of the extent to which species characteristics were phylogenetically related to range shifts at the contracting (trailing edge) and expanding (leading edge) limits. We show that species shifts at both range limits are related to different combinations of traits and exhibit different phylogenetic correlation patterns, bringing novel evidence that divergent mechanisms underlie how species are responding to current climate changes by shifting their ranges. Overall, our findings suggest that trait-based approaches coupled with phylogenetic information may offer a simple way to help predict species vulnerability to future climate change. Phylogenetic signal When considering binary responses, range shifts at the lower altitudinal limit were phylogenetically conserved ( D =0.26, P =0.022, permutation test, n =1,000), indicating that species contracting their range at their trailing edge were more closely related than would be expected by chance ( Fig. 2 ). Reconstruction of ancestral states along the phylogeny also indicated a strong in-depth phylogenetic clustering in both the binary and continuous climate-induced range shifts at the trailing edge, although the latter was not significant when tested at the final nodes ( Fig. 3 ). In contrast, shifts in the upper altitudinal limit (that is, colonization of newly suitable habitats) were not phylogenetically clustered when considering either binary ( D =1.24, P =0.794, permutation test, n =1,000; Fig. 2 ) or continuous responses ( Fig. 3 ). Our conclusions regarding the significance of phylogenetic clustering in shifters versus non-shifters were robust to variation in tree topology as we found only slight variation in the D values and associated tests over the 100 trees selected at random from the posterior distribution of trees (lower limit: D =0.28±0.03 s.d., P =0.007–0.029, permutation test, n =1,000; upper limit: D =1.22±0.04 s.d., P =0.633−0.823, permutation test, n =1,000). 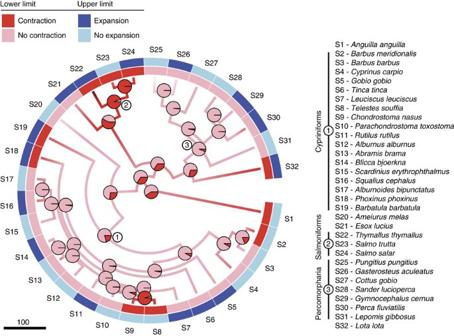Figure 2: Phylogenetic clustering of climate-induced range shift. Maximum clade credibility tree of 32 freshwater fish species depicting climate-induced range shifts in lower and upper altitudinal limits. Rates of range shifts were first controlled for the effects of extrinsic drivers and then converted into binary response variables indicating whether the range limit had move upslope (contraction or expansion; value=1) or not (value=0), as illustrated at the final nodes by dark and light colours, respectively. Pies indicate the frequencies of the marginal ancestral state reconstructions of the binary variable depicting climate-induced range shifts in lower limit at the internal nodes of the tree. Branch colours indicate ancestral state reconstructions of the rate of climate-induced shifts in lower altitudinal limit along the edges and internal nodes of the tree, with dark colours indicating the stronger shifts. The scale bar indicates the divergence time estimates for the phylogenetic reconstruction in millions of years before present. Figure 2: Phylogenetic clustering of climate-induced range shift. Maximum clade credibility tree of 32 freshwater fish species depicting climate-induced range shifts in lower and upper altitudinal limits. Rates of range shifts were first controlled for the effects of extrinsic drivers and then converted into binary response variables indicating whether the range limit had move upslope (contraction or expansion; value=1) or not (value=0), as illustrated at the final nodes by dark and light colours, respectively. Pies indicate the frequencies of the marginal ancestral state reconstructions of the binary variable depicting climate-induced range shifts in lower limit at the internal nodes of the tree. Branch colours indicate ancestral state reconstructions of the rate of climate-induced shifts in lower altitudinal limit along the edges and internal nodes of the tree, with dark colours indicating the stronger shifts. The scale bar indicates the divergence time estimates for the phylogenetic reconstruction in millions of years before present. 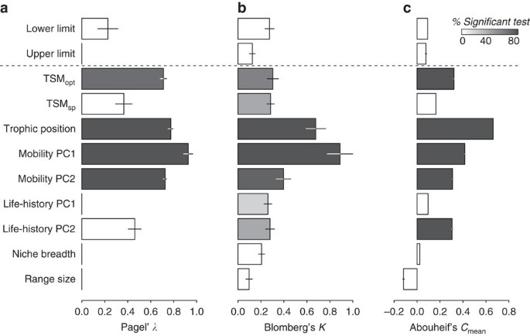Figure 3: Phylogenetic signal in range shifts and species traits. Phylogenetic signal indices and tests in rates of range shifts and species traits for 32 freshwater fish species calculated over 100 trees selected at random from the post-burn-in MCMC search of the parameter space during phylogenetic reconstruction: (a) Pagel’sλ, (b) Blomberg’sKand (c) Abouheif’sCmean. Bars are s.d. across the 100 phylogenetic trees. Grey scale indicates the percentage of associated significant (P<0.05) tests over the 100 trees. Full size image Figure 3: Phylogenetic signal in range shifts and species traits. Phylogenetic signal indices and tests in rates of range shifts and species traits for 32 freshwater fish species calculated over 100 trees selected at random from the post-burn-in MCMC search of the parameter space during phylogenetic reconstruction: ( a ) Pagel’s λ , ( b ) Blomberg’s K and ( c ) Abouheif’s C mean . Bars are s.d. across the 100 phylogenetic trees. Grey scale indicates the percentage of associated significant ( P <0.05) tests over the 100 trees. Full size image Similarly, species characteristics displayed different levels of phylogenetic signal, with the three indices leading to consistent results ( Fig. 3 ). For instance, traits related to morphological attributes (for example, mobility PC1) or trophic position showed strong phylogenetic clustering, while those related to life-history characteristics and specialization (for example, niche breadth) were more evolutionary labile. Although thermal tolerances per se showed a strong phylogenetic signal, with λ values for T opt and T sp of 0.76 (±0.02 s.d.) and 0.63 (±0.10 s.d. ), respectively, measures of thermal safety margins appeared to be less linked to phylogenetic relatedness, especially when considering the optimal spawning temperature (TSM sp ; Fig. 3 ). Relationships between range shifts and species traits As expected, the physiological sensitivity of species through their capacity to tolerate further warming (TSM opt ) had a preponderant and negative effect on the rate of retreat of the lower altitudinal limit ( Fig. 4a ; Table 1 ). Species with smaller thermal safety margins (that is, those with lower T opt relative to climate means) have suffered more from local extinctions at their trailing edge than species with higher thermal safety margins. Although this relationship seemed underlined by strong phylogenetic constraints existing on their thermal tolerances, the phylogenetic clustering of range retreat was further complicated by high variability in responses among species when considering the continuous rates of shifts, as outlined by the branches crossing within the phylogenetic traitgram ( Fig. 5a ). Interestingly, the trophic position appeared to be a strong predictor of shifts at the leading edge, with piscivorous species showing higher rates of expansion ( Fig. 4b ; Table 1 ). These shifts were also strongly influenced by life-history strategies of species, which, contrarily to the trophic position, showed a weak phylogenetic signal ( Fig. 3 ). Species with high propagule pressure (that is, r -strategists, life-history PC2) displayed the greatest shifts without this being apparently influenced by phylogenetic constraints. Nonetheless, this relationship appeared further blurred by the influence of other characteristics, as outlined by the criss-crossing of colours along the internal branches of the tree ( Fig. 5b ). Finally, shifts were also related, albeit weakly, to mobility PC1 and TSM opt . Overall, all the selected models explained non-trivial amounts of variability in climate-induced range shifts at both contracting and expanding limits ( R 2 =0.23–0.38; Table 1 ). 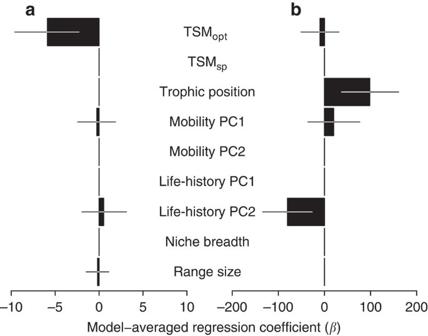Figure 4: Results of model-averaging for models relating range shifts to species traits. Model-averaged slope regression coefficients standardized toz-scores for phylogenetic generalized least squares relating shifts at (a) the lower and (b) the upper altitudinal limit to species traits for 32 freshwater fish species. Bars are 95% confidence interval. High values of mobility PC1 and mobility PC2 indicate a greater mobility at larval and adult stages, respectively. High values of life-history PC1 and small values of life-history PC2 indicate a greater propagule pressure. Figure 4: Results of model-averaging for models relating range shifts to species traits. Model-averaged slope regression coefficients standardized to z -scores for phylogenetic generalized least squares relating shifts at ( a ) the lower and ( b ) the upper altitudinal limit to species traits for 32 freshwater fish species. Bars are 95% confidence interval. High values of mobility PC1 and mobility PC2 indicate a greater mobility at larval and adult stages, respectively. High values of life-history PC1 and small values of life-history PC2 indicate a greater propagule pressure. Full size image Table 1 Results of model selection for models relating range shifts to species traits. 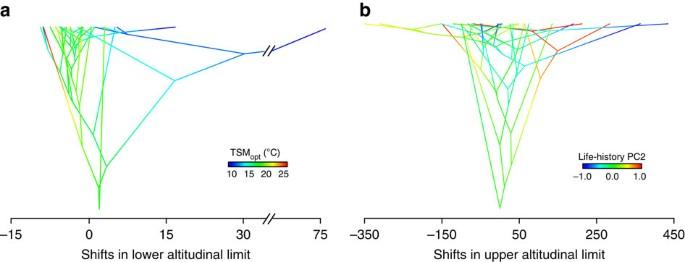Figure 5: Underlying phylogenetic relatedness between range shifts and species traits. Traitgrams depicting the relationships between the rates of climate-induced range shifts at (a) the lower and (b) the upper altitudinal limit (xaxis) and their underlying phylogenetic relatedness (time from the root;yaxis) using the maximum clade credibility tree for 32 freshwater fish species. A high level of branches crossing indicates convergent evolution across clades and weak phylogenetic signal. Rates of climate-induced range shifts were controlled for the effect of extrinsic drivers and expressed as the residuals of the linear regression linking the range shifts to the potential confounders. Colours indicate ancestral state reconstructions of (a) the species capacity to tolerate further warming (TSMopt) and (b) the propagule pressure (life-history PC2), along the edges and internal nodes of the tree: blue indicates small values and red high values. Small values of life-history PC2 indicate a greater propagule pressure. Full size table Figure 5: Underlying phylogenetic relatedness between range shifts and species traits. Traitgrams depicting the relationships between the rates of climate-induced range shifts at ( a ) the lower and ( b ) the upper altitudinal limit ( x axis) and their underlying phylogenetic relatedness (time from the root; y axis) using the maximum clade credibility tree for 32 freshwater fish species. A high level of branches crossing indicates convergent evolution across clades and weak phylogenetic signal. Rates of climate-induced range shifts were controlled for the effect of extrinsic drivers and expressed as the residuals of the linear regression linking the range shifts to the potential confounders. Colours indicate ancestral state reconstructions of ( a ) the species capacity to tolerate further warming (TSM opt ) and ( b ) the propagule pressure (life-history PC2), along the edges and internal nodes of the tree: blue indicates small values and red high values. Small values of life-history PC2 indicate a greater propagule pressure. Full size image Changes in species distributions are multifaceted and complex [30] , and disentangling the underlying mechanisms driving these range shifts has proven to be difficult [16] . Here, we provide novel evidence that dissimilar mechanisms may underlie how species are responding to current climate changes by shifting their ranges. We demonstrate that range shifts are related to shared ecological characteristics ( Fig. 4 ; Table 1 ), which is consistent with theoretical expectations about species abilities to cope with climate change [6] , [31] , [32] , but that these underlying mechanisms are differentially related to phylogeny ( Figs 2 and 3 ). Our findings support the hypothesis that, to a large extent, the capacity of species to tolerate further warming, a highly phylogenetically conserved trait, determines range contractions at the trailing edge. In contrast, range expansions at the leading edge are related to a combination of species attributes linked to their intrinsic sensitivity, but also to their resilience ability to track optimal conditions. In particular, more evolutionarily labile life-history characteristics related to species dispersal ability appear especially important to explain upslope colonization. This study highlights that assessing vulnerability of species to climate change requires to consider diverse facets of species responses, a framework that has already been called for [8] , [16] . It also demonstrates that exploring the relationships between species responses and species traits in light of species evolutionary history may unravel the underlying determinants of species responses to climate change. To date, testing simple relationships between range shifts and species traits has not been a successful approach in elucidating the mechanistic causes of range dynamics during climate warming [7] , [33] , [34] . Given that the response of species depends on regional patterns of exposure to climate change [31] , [34] , our methodological framework controlling for these effects could help to disentangle these mechanisms [19] . Nonetheless, the failure of most empirical studies to identify a clear relationship between species range shifts and their traits may stem from inconsistencies in the way range shifts are assessed (that is, changes in range size [35] , range centre [33] , warm limit [36] , [37] or cold limit [18] ). As a result, the lack of consensus has previously been suggested to result from different mechanisms acting at opposite ends of species distributions but considered without distinction [7] . Our results strongly support this contention, revealing the importance of studying the dynamics of both contracting and expanding limits. Shifts at the trailing edge provide some support for phylogenetic conservatism ( Fig. 2 ). They correlate with species thermal safety margins ( Fig. 4 ; Table 1 ), a measure likely to reflect the direct influence of climate change [23] , [25] displaying a strong phylogenetic signal ( Fig. 3 ). This phylogenetically selective pattern of extinctions is in line with both palaeontological observations and predictions, suggesting that species losses may not be randomly distributed across the tree of life [5] , [32] . As local extirpations drive the global extinction of species [6] , the phylogenetic non-randomness in range contraction derived from comparing shifters versus non-shifters suggests that the evolutionary history of species may be an important determinant of extinction risk. The generality of our finding is strengthened by concordant range contractions observed for thermal sensitive macroinvertebrates in Australia [17] and lizards in Mexico [21] . This pattern supports the assertion that species living closer to their thermal limits are likely to face increased extinction risk as they cannot evolve physiological tolerances rapidly enough to cope with climate change due to evolutionary constraints on their thermal tolerance [3] , [4] , [21] . Nevertheless, although the presence or absence of climate-induced range shifts were generally more similar between closely related species, the strength of this phylogenetic signal was weak when considering the continuous rates of shifts ( Figs 3 and 5 ). Unravelling phylogenetic signal in small phylogenies has proven to be difficult, even under strong phylogenetic clustering [38] . This pattern also suggests that beyond methodological uncertainties, extinction selectivity may in fact be obscured by the influence of fine-scale environment. Here, air temperature was used as a surrogate of water temperature, and although both are strongly related [39] , incorporating information on microclimates may be central to providing more accurate estimates of thermal sensitivity of species and ultimately distribution shifts [23] , [40] . In contrast to the trailing edge analyses, lack of phylogenetic clustering in range shifts at the leading edge ( Figs 2 , 3 and 5 ) largely reflects the fact that ecological traits promoting colonization abilities are not shared by close relatives ( Fig. 4 ; Table 1 ). This may suggest that strong environmental filters have favoured convergence for similar traits involved in climate tracking for species in distant clades. In particular, we found that species expanding their range tend to be fast developing and so better equipped for coping with habitat instability [41] . Several studies have identified a similar correlation [36] , [37] , [42] . However, whether these relationships hold between latitudinal and elevation gradient is still unclear [34] , [42] . Given the apparent lability of these traits, our results suggest that on expanding range limits, evolutionary changes in life-history traits might arise and accelerate range expansion [27] . Despite the fact that direct evidence of genetically based adaptation to climate change over time remains sparse, the contribution of rapid evolution to range expansion has already been observed in insects and plants, disrupting the separation of ecological and evolutionary time scales [43] , [44] . Evidence from palaeoecology also suggests that establishing new ranges as the climate changes involves a great deal more than the dispersal of a propagule ahead of the advancing species front [9] . Here, we demonstrate that trophic position is of uttermost relevance in determining the current rate of range expansion. These results might support to a certain extent—albeit indirectly—that changing species interactions may have an even greater role than physiological tolerance to high temperatures in climate change impacts [12] . However, they may also reflect the influence of other species characteristics, for instance dispersal ability—the highest-trophic-level species are generally also the largest ones—all things being equal. The mechanisms identified here provide an informed but incomplete vision of how species respond to climate change by shifting their ranges. The dynamics of range shifts is further structured by the spatial distribution of suitable habitats, which is often patchy (naturally or anthropogenically fragmented [45] ) and can lead to differential time lags in climate tracking [1] . This is especially true in freshwater ecosystems where the directionality of water flows and the presence of physical barriers can restrict the redistribution of species under changing climate [46] . Changes in other confounding factors as well as the spatiotemporal variability in climate may also help to enhance our ability to predict range shifts [35] , [40] . The predictive science of range shifts would thus greatly benefit from coupling species characteristics with extrinsic factors such as the spatial distribution and availability of habitats [47] . In addition, mechanisms underlying shifts in latitude and elevation may not be equivalent, which underscores the need to develop a comprehensive framework to assess multidimensional changes in species distributions [16] , [42] . The lower performance of models predicting the magnitude of range contractions compared with that of range expansions also raises the possibility of other response mechanisms to climate change. Linking range shift patterns among multiple species to their intrinsic characteristics has proven to be a tricky task when considering range retreats, as suggested by the lack of [18] or the weak [34] relationships previously documented. Along with shifts in range limits, phenology is likely to be influenced by a rise in temperature which can potentially drive phylogenetically-biased patterns of species loss [19] . Similarly, behavioural plasticity could also be a crucial mechanism for species to avoid heat stress [22] , [23] , possibly underlined to some extent by phylogenetic constraints [48] . Thus, although the best explanation of trailing edge retreat is underpinned by the physiological capacity of species to tolerate further warming, other traits linked to their resilience ability might also contribute to the pattern of phylogenetic selectivity in extinction. Importantly, the generalization of the contribution of these mechanisms to the phylogenetic selectivity in extinction could be challenged since acclimation and behavioural regulation can substantially vary among lineages [23] , [48] , while the warming tolerance of aquatic organisms is strongly dependant on oxygen-limited thermal tolerance [20] . Therefore, although our general conclusions would remain unaltered, these results point towards the critical need to find out whether other extrinsic and intrinsic factors may be contributing to, rather than blurring, the phylogenetic pattern of extinction documented here. Finally, our results, combined with those of previous studies [5] , [19] prove that phylogenetic history provides useful insights into how species and communities are likely to respond to future climate change. The use of phylogenies to predict species vulnerability may provide a simple way to integrate species differences across multiple traits in conservation assessments [49] to prioritize taxa with the greatest potential vulnerability, while simultaneously considering their phylogenetic uniqueness in conservation decisions [6] , [50] , [51] . To make progress in this field, further work is required to overcome the difficulty in establishing general mechanisms for biological responses to climate change [16] . Nonetheless, we also demonstrate that phylogeny poorly predicted range expansion. These findings emphasize how combining trait-based and phylogenetic approaches may offer new opportunities in facing conservation challenges. In the near future, biodiversity patterns could be greatly modified owing to the spatially selective reshuffling of communities with species displaying specific combinations of traits and evolutionary history. Whether the biological impacts of climate change will ultimately depend on the complex interplay of species responses thus deserves urgent attention. Only with improved understanding of the potential impacts of species range shifts on biological interactions and their consequences on ecosystem functioning will researchers be able to quantify the ecological threat posed by future climate change. Species range shifts To identify the mechanisms involved in climate-induced species range shifts, we used shifts at the lower (that is, trailing edge) and upper (that is, leading edge) altitudinal limits previously documented for 32 species of stream fish in France over two periods of time (1980–1992 and 2003–2009) (ref. 52 ). This study identified systematic range shifts for most species towards higher altitudes, which were consistent with geographic variations in climate change velocities observed across the French hydrographic network, thus providing strong support that stream fish are currently tracking ongoing climate warming. Range shifts were reported as mean rates of displacement towards higher elevations in meters, based on spatial distributions described using species distribution models (see Supplementary Methods ; Supplementary Figs 1 and 2 ). More specifically, species ranges were mapped at the scale of stream reaches (that is, 2 km lengths) throughout the whole French hydrographic network for each time period and each species using an ensemble modelling approach combining several modelling and threshold-setting methods ( Fig. 6 ). On the basis of these maps, the lower and upper range limits were defined as the 2.5 and 97.5%, respectively, of the altitudes where the species were predicted to be present. All models demonstrated high predictive performances, with a mean area under the curve value of 0.88 (±0.05 s.d.). In addition, no link was found between variations in species detectability and distribution changes over time. To determine the rate of shift, linear regressions were then fitted for each species between the measures of range limits (that is, upper or lower limit) and the time period from which the range limit was estimated. To adjust for the effect of methodological choices in estimating species range limits, the threshold-setting method was added into the model as a confounding variable and the shifts estimated by the regression coefficient of the period-group effect (that is, defining how much the range limit changed in the 2003–2009 period after adjusting for the potential methodological confounder; see Supplementary Methods ; Supplementary Fig. 3 for details). 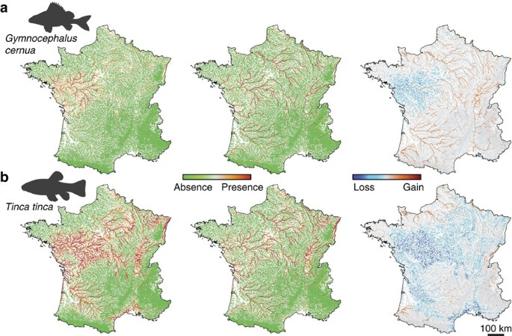Figure 6: Examples of distribution shifts across the French hydrographic network. Maps for two species with contrasted responses: (a)Gymnocephalus cernuaand (b)Tinca tincashowing the spatial distribution in the 1980–1992 period (left panel) and 2003–2009 period (middle panel). The agreement between presence and absence predictions was measured by summing the 90 predictions (iterations × threshold-setting methods) for each reach of the hydrographic network, with a colour scale ranging from green (no predicted presence) to red (90 predicted presences). Differences in occurrence between the two time periods (right panel) with a colour scale ranging from blue for a loss of suitable habitat (90 presences predicted only for the 1980–1992 period) to red for a gain in suitable habitat (90 presences predicted only for the 2003–2009 period). Figure 6: Examples of distribution shifts across the French hydrographic network. Maps for two species with contrasted responses: ( a ) Gymnocephalus cernua and ( b ) Tinca tinca showing the spatial distribution in the 1980–1992 period (left panel) and 2003–2009 period (middle panel). The agreement between presence and absence predictions was measured by summing the 90 predictions (iterations × threshold-setting methods) for each reach of the hydrographic network, with a colour scale ranging from green (no predicted presence) to red (90 predicted presences). Differences in occurrence between the two time periods (right panel) with a colour scale ranging from blue for a loss of suitable habitat (90 presences predicted only for the 1980–1992 period) to red for a gain in suitable habitat (90 presences predicted only for the 2003–2009 period). Full size image Although almost all species studied are widely distributed in Europe, the French climate delineates the warm limit for most, enabling the mechanisms underlying their responses to climate change to be studied at both ends of their distribution along the altitudinal gradient defined across France ( Supplementary Methods ; Supplementary Figs 4–6 ). However, to control for effects of confounding factors likely to influence species range shifts, the range shift measures were first regressed against two covariates: degree of exposure to climate change, estimated as mean climate change velocities experienced by a species at its lower or upper altitudinal limit, and degree of anthropogenic manipulation, estimated through an index of popularity of the species in France, assuming that the most popular species would be more likely to be manipulated through use in aquaculture, as bait or as gamefish (see Supplementary Table 1 for details on confounding variables). As some species may occupy areas where climate has changed faster, they should not all be expected to shift upslope at the same rate. Controlling for the velocity of climate change allows the pace and direction of climate change to be described and thus to provide improved expectations for range shifts [1] , [53] . In addition, human commercial or recreational activities may give species more opportunity to move into previously unsuitable habitats (that is, human-mediated dispersal), leading to range expansions, or conversely reduce species persistence (that is, human-induced species loss), leading to range contraction [54] . Although the degree of human manipulation was not related to species range shifts along the altitudinal gradient, as expected the velocity of climate change explained a non-trivial amount of variability in range shifts, especially at the upper limit (lower: R 2 =0.045, Supplementary Table 2 ; upper: R 2 =0.291, Supplementary Table 3 ). Regression residuals were then used in all subsequent analyses as estimates of the relative rates of climate-induced range shifts at both the lower and upper altitudinal limits, adjusted for the effects of climatic and non-climatic extrinsic factors. Species traits We initially selected 16 different traits to test our theoretical expectations ( Fig. 1 )—(see Supplementary Table 4 for details). As temperature can act as a stress inhibitor by affecting several different functions, we used two thermal tolerance traits derived from response fitness curves measured in laboratory experiments: the upper limit of the optimal temperature range ( T opt ), defined as the range over which feeding occurs and there are no external signs of abnormal behaviour and the optimal spawning temperature ( T sp ). However, although thermal performance curves describe the direct effect of temperature on organism fitness, the fitness impacts of warming at each location also depend on the optimal temperature position relative to the local climate [24] , [25] . Therefore, we did not use thermal tolerance per se , but the difference between the thermal tolerances ( T opt , T sp ) and the thermal habitat of species ( T hab ), here taken to be mean annual water temperature in the initial period. These measures approximate the average amount of temperature increase that species can tolerate before performance drops, namely the thermal safety margin [25] : TSM opt and TSM sp (see Supplementary Fig. 7 for details). The trophic position was defined as herbivorous, omnivorous, invertivorous, invertivorous-carnivorous to piscivorous. Despite being difficult to estimate directly, the ability of species to disperse is often estimated for actively dispersing organisms from their morphological characteristics [55] . In particular, body size is closely correlated with the greatest dispersal distance an active disperser is able to achieve [56] . We therefore included two traits related to body size: that in adults (body length) and that in larvae (larval length) and two ratios describing the hydrodynamic profile of the fish (shape factor) and their capacity for sustained swimming (swimming factor). Collinearity between these traits was reduced using a principal co-ordinates analysis and mobility was summarized by the first two axes. The first axis (mobility PC1) was interpreted as larval mobility, and the second (mobility PC2) as adult mobility (that is, high values of mobility PC1 and mobility PC2 indicate a greater mobility, Supplementary Table 5 ). As the ratios had very skewed distributions, they were log-transformed before the analysis. We used seven traits related to life-history: female fecundity (number of oocytes), spawn time, egg diameter at hatching, life span, female maturity, length of incubation period and parental care. We then used the first two axes of a principal co-ordinates analysis to summarize these seven traits, the first axis (life-history PC1) being positively correlated to propagule pressure and describing the rate of population turnover (that is, high values indicate a greater fecundity and life cycle duration) and the second (life-history PC2) being negatively correlated to propagule pressure and describing the position of the species along the r - K continuum (that is, small values indicate a greater reproductive capacity and development time, Supplementary Table 5 ). To describe environmental specialization, we used the outlying mean index analysis [57] to estimate the niche breadth, calculated as s.d. of environmental space used by each species in the initial period along the main axes of the outlying mean index, including three environmental variables (slope, elevation and upstream–downstream position). This niche axis was considered to reflect the tolerance of a wide range of abiotic conditions, including climatic factors and was therefore interpreted as habitat generalization as well as thermal generalization. Range size was estimated as percentage of total network length predicted to be occupied by the species in the initial period. Overall, this led us to keep nine variables summarizing species characteristics. Although dependence of thermal tolerance on physiology could lead to interdependence of several of these traits, the variance inflation factors were less than 1.45, indicating that there were no problems with multicollinearity among the predictors in the models. Phylogeny We used a dated phylogeny reconstructed from complete mitochondrial genomes on 151 Teleostei fish using Bayesian inference as our phylogenetic hypothesis (see Supplementary Methods ; Supplementary Fig. 8 ; Supplementary Tables 6 and 7 for details). Species were pruned from this tree so as to keep only the 32 species for which range shift information was available. Nevertheless, to assess the effect of phylogeny reconstruction on the robustness of our results, all statistical analyses were conducted on 100 trees selected at random from the post-burn-in MCMC search of the parameter space. Phylogenetic signal The phylogenetic signal, meaning the tendency of closely related species to share more similar values than species drawn at random from the tree [28] , was evaluated using different indices, as this selection could lead to contrasted results [38] . Pagel’s λ [58] , Blomberg’s K [29] and Abouheif’s C mean [59] and their associated tests were first used to test the phylogenetic signal in the relative rates of climate-induced range shifts at both altitudinal limits as well as in species attributes. These indices are considered statistically powerful for measuring whether data exhibit phylogenetic signal and, although they do not have the same properties, stronger deviations from zero indicate stronger relationships between species characteristics and the phylogeny. Under a Brownian motion model, where species inherit their traits from ancestors but then slowly diverge by small random amounts and at a constant rate through time, Pagel’s λ and Blomberg’s K are expected to be equal to 1. Alternatively, λ or ϰ values of 0 imply that there is no phylogenetic dependence, while 0< λ or ϰ <1 correspond to some degree of trait lability. In contrast, Abouheif’s C mean is an index which is not based on an evolutionary model, but designed to test phylogenetic autocorrelation. However, as the statistical power of detecting significant trends in range shifts may be obscured by the use of continuous estimates of range shift rates, we also tested the phylogenetic signal on binary comparisons of shifters versus non-shifters. To that end, we converted the shift rates at both range limits into binary response variables indicating whether the range limit had expanded or contracted upslope (value=1) or not (value=0). The phylogenetic signal was then estimated by the D value, expressed as the sum of changes in estimated nodal values of the binary variable along the edges of the phylogeny [60] . If shifts are highly phylogenetically clustered, D value will be 0, while if the shifts are more labile, D will be higher. The distribution of the null expectation of D under no phylogenetic signal obtained by randomly shuffling the tips of the phylogeny 1,000 times was then used to test the significance of the observed D value. Finally, to visualize how range shifts varied with phylogenetic depth, we reconstructed the ancestral states in both rates of climate-induced range shifts and their binary outputs along the internal nodes and edges of the tree. Continuous shift rates were reconstructed using a fast estimation of maximum likelihood ancestral states at internal nodes and a fractional method allowing to interpolate the state estimates along the edges of the phylogeny [61] . Reconstruction of binary comparisons of shifters versus non-shifters was estimated by a rerooting method [62] , which estimates the marginal ancestral state for each internal node of the tree using likelihood and assuming an equal rate of evolution. Relationships between range shifts and species traits Expected relationships between rates of range shifts and species attributes were tested using phylogenetic generalized least squares (PGLS). This method allows to account for data non-independence by adjusting the variance/covariance matrix to the phylogenetic relatedness among species using Pagel’s λ according to processes other than pure Brownian motion [58] . All predictors were transformed to z -scores to standardize slope coefficients ( β ) to compare the relative strength of the predictors. We constructed all combinations of models for a maximum of three out of the nine final variables, in accordance with the general rule of thumb limiting the number of predictors to one-tenth of the number of observations (that is, 32 species). We used the Akaike information criterion adjusted for small sample size (AICc) for multimodel inference [63] . We performed model averaging accounting for model uncertainty using a conservative method by averaging the slope coefficients ( β ) across all models with ΔAICc ≤2 from the model with the lowest AICc, using Akaike weights ( w i ), and including zeros when predictors did not occur in a particular model. To assess the robustness of our results according to phylogenetic uncertainty, multimodel inference was performed on all combinations of models run with each of the 100 phylogenetic tree randomly selected from the Bayesian posterior distribution of trees (that is, 13,000 models). However, similar results were obtained when the maximum clade credibility tree was considered as the only phylogenetic hypothesis ( Supplementary Fig. 9 ; Supplementary Table 8 ). Models and analyses were developed using R environment software v 2.13.0 (ref. 64 ) using ape, picante, nlme and phytools packages. How to cite this article: Comte, L. et al. Species traits and phylogenetic conservatism of climate-induced range shifts in stream fishes. Nat. Commun. 5:5053 doi: 10.1038/ncomms6053 (2014).